A universal critical density underlying the physics of electrons at the LaAlO3/SrTiO3interface The two-dimensional electron system at the interface between the insulating oxides LaAlO 3 and SrTiO 3 exhibits ferromagnetism, superconductivity and a range of unique magnetotransport properties. An open experimental challenge is to identify, out of the multitudinous energy bands predicted to exist at the interface, the key ingredients underlying its emergent transport phenomena. Here we show, using magnetotransport measurements, that a universal Lifshitz transition between d orbitals of different symmetries lies at the core of the observed phenomena. We find that LaAlO 3 /SrTiO 3 systems generically switch from one- to two-carrier transport at a universal carrier density, which is independent of the LaAlO 3 thickness and electron mobility. Interestingly, the maximum superconducting critical temperature occurs also at the Lifshitz density, indicating a possible connection between the two phenomena. A simple band model, allowing for spin-orbit coupling at the atomic level, connects the observed transition to a variety of previously reported properties. Our results demonstrate that the fascinating behaviour observed so far in these oxides follows from a small but fundamental set of bands. A key feature of the electron gas at the LaAlO 3 /SrTiO 3 (LAO/STO) interface [1] is that its ground state can be tuned using field-effect gating [2] . Ferromagnetic [3] , [4] and superconducting [5] , [6] ground states have been demonstrated in this system, as well as their coexistence [7] , [8] , [9] . Superconductivity was shown to emerge at a certain gate voltage, concomitant with the appearance of strong spin–orbit (SO) interactions [10] . At higher gate voltages, the critical temperature of superconductivity was shown to slowly decrease [6] , [11] together with a similar decrease in SO strength [12] . A growing body of theoretical works [13] , [14] , [15] , [16] , [17] predict that at the interface there would be a large number of electronic sub-bands, suggesting that the above transport characteristics might be rather sensitive to the details of the disorder and of the confining potential at the interface. This complexity is further supported by transport [11] , [18] , [19] , [20] , optical [21] and heat conductivity [22] measurements that proposed that at high-carrier densities this system has multiple types of carriers existing at different distances from the interface, possibly on different TiO 2 planes [11] , [13] , [14] , [17] , [21] , [23] . Thus, to date, a simple relation between specific energy bands and the fundamental transport phenomena observed in this system is still missing. In this paper, we show using magnetotransport experiments that the physics at the interface follows from a universal picture with a minimal number of energy bands, implying that only a few among the manifold of states are important. Specifically, we show that a variety of behaviour of this two-dimensional (2D) system can be traced back to a special point where the system undergoes a Lifshitz transition between populations of d orbitals of different symmetries. Observation of a special point in transport of LAO/STO system All measured LAO/STO samples showed a critical gate voltage across which their transport characteristics changed significantly. We have measured four samples differing in their LAO layer thickness and spanning an order of magnitude in mobility, all showing similar behaviour. 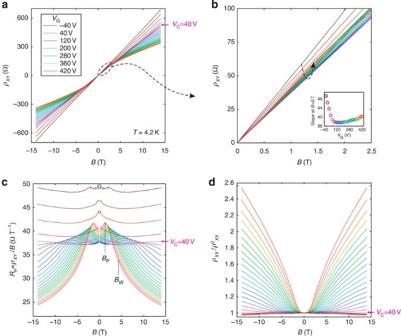Figure 1: Observation of a critical transition in transport at the LAO/STO interface. (a) Measured Hall resistance,ρXY, versus magnetic field,B, for various back-gate voltages,VG, in 20 V steps, atT=4.2 K. At a critical value,VC=40 V, a transition is observed between two different types ofBdependencies. (b) Zoom-in on the low-field region of (a). The low-field slopes reverse their gate dependence atVC(inset): belowVCthey decrease with increasing gate-voltage, they saturate nearVC, and then slightly increase. (c) Corresponding Hall coefficient,RH=ρXY/B, plotted versusBfor the sameVG's as in (a). BelowVC,RHis roughly independent ofB, but aboveVCit peaks at an intermediate field and falls off at high fields. Indicated for the highestVGis the position of the peak,Bp, and the falloff field,BW, which is determined from the deflection point of the curve. These characteristic fields depend onVG. (d) Measured longitudinal resistivity,ρXX, normalized by its value atB=0,ρ0XX, plotted as a function ofBfor the sameVG's as in (a). Figure 1a shows the measured ρ XY as a function of magnetic field, B , at various gate voltages for sample 1. Starting from the lowest gate voltage V G =−40 V and up to a critical value V C =40 V, ρ XY is linear in B with a slope that decreases with increasing V G . This behaviour is expected from the field-effect tuning of carrier density. However, as we cross V C the shape of the Hall traces changes considerably; they become kinked, with the kink position progressively moving to lower B with increasing V G . Zooming-in on the low-field Hall slopes ( Fig. 1b ) we find that they too undergo a significant change at V C , from slopes that gradually decrease with increasing V G below V C , to slopes that are roughly constant and even slightly increasing above V C (inset Fig. 1b ). Thus, both the low- and high-field Hall characteristics signify that a distinct transition occurs in the system at V C . Figure 1: Observation of a critical transition in transport at the LAO/STO interface. ( a ) Measured Hall resistance, ρ XY , versus magnetic field, B , for various back-gate voltages, V G , in 20 V steps, at T =4.2 K. At a critical value, V C =40 V, a transition is observed between two different types of B dependencies. ( b ) Zoom-in on the low-field region of ( a ). The low-field slopes reverse their gate dependence at V C (inset): below V C they decrease with increasing gate-voltage, they saturate near V C , and then slightly increase. ( c ) Corresponding Hall coefficient, R H = ρ XY / B , plotted versus B for the same V G 's as in ( a ). Below V C , R H is roughly independent of B , but above V C it peaks at an intermediate field and falls off at high fields. Indicated for the highest V G is the position of the peak, B p , and the falloff field, B W , which is determined from the deflection point of the curve. These characteristic fields depend on V G . ( d ) Measured longitudinal resistivity, ρ XX , normalized by its value at B =0, ρ0 XX , plotted as a function of B for the same V G 's as in ( a ). Full size image This transition becomes even more striking when we plot the Hall coefficient R H = ρ XY / B as a function of B and V G ( Fig. 1c ). Below V C , R H is roughly a constant as a function of B , whose value decreases with increasing V G . Above V C , however, the curves acquire a qualitatively different form: they first increase with field at low fields, then peak at an intermediate field, B p , (see Supplementary Methods for more details about this peak) and finally drop down at high fields yielding an overall bell-like shape, whose width we define as B W ( Fig. 1c caption). The characteristic field, B W , progressively decreases as V G is increased. This trend in R H is echoed by the longitudinal resistance, ρ XX ( Fig. 1d ). Below V C , ρ XX is practically independent of B , but above V C , ρ XX remains flat only up to an intermediate characteristic field after which it rises continuously. Just like B W , this characteristic field becomes smaller with increasing V G . The self-similarity of the transport traces on each side of the transition point suggests that they can be grouped into two generic forms. Below V C , the curves have almost identical shapes up to an offset ( Fig. 2a,b ). Above V C , the curves ( Fig. 1c,d ) differ substantially in their dependence on B . However, if for every gate voltage we add a y-offset, scale the curve height and plot it as a function of the scaled magnetic field, B / B W , we observe that all R H curves perfectly collapse onto a single trace ( Fig. 2c ). This suggests that the Hall resistance above V C is described by a generic functional form. Interestingly, if we use the field with which we scaled R H to scale the ρ XX trace at the same gate voltage, we find that all the ρ XX traces also collapse perfectly ( Fig. 2d ). The fact that ρ XY and ρ XX scale together demonstrates their strong connection. 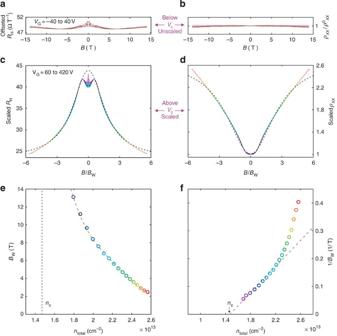Figure 2: Scaling of transport curves above and below the critical gate voltageVC. The curves inFig. 1c,dseparate into two groups, which scale differently. (a) BelowVC, theRHtraces merge by a mere shift along theyaxis. (b) The normalizedρXXcurves belowVCare already self-similar. (c) AboveVC, theRHcurves differ substantially in their characteristic fields, but when plotted versusBdivided by the characteristic width,B/BW, after subtracting a y-offset and scaling of their height, all of them collapse perfectly. Lorentzian fit (dashed line). (d) TheρXXcurves aboveVC, plotted as a function ofB/BW, whereBWis taken from theRHcurve at the same gate voltage. This scaling yields perfect collapse also of theρXXtraces, showing the strong correlation betweenρXXandRH. Lorentzian fit (dashed line) (e)BWplotted versus carrier density,ntotal, obtained from the high-field Hall data (the grey dashed line is a guide to the eye).BWseems to diverge at a critical density,nC. (f) This critical density is estimated from thex-intercept of the plot of the inverse field, 1/BW, versus density (the dashed line is a linear fit to the low-density data). Figure 2: Scaling of transport curves above and below the critical gate voltage V C . The curves in Fig. 1c,d separate into two groups, which scale differently. ( a ) Below V C , the R H traces merge by a mere shift along the y axis. ( b ) The normalized ρ XX curves below V C are already self-similar. ( c ) Above V C , the R H curves differ substantially in their characteristic fields, but when plotted versus B divided by the characteristic width, B/B W , after subtracting a y-offset and scaling of their height, all of them collapse perfectly. Lorentzian fit (dashed line). ( d ) The ρ XX curves above V C , plotted as a function of B/B W , where B W is taken from the R H curve at the same gate voltage. This scaling yields perfect collapse also of the ρ XX traces, showing the strong correlation between ρ XX and R H . Lorentzian fit (dashed line) ( e ) B W plotted versus carrier density, n total , obtained from the high-field Hall data (the grey dashed line is a guide to the eye). B W seems to diverge at a critical density, n C . ( f ) This critical density is estimated from the x -intercept of the plot of the inverse field, 1/ B W , versus density (the dashed line is a linear fit to the low-density data). Full size image In Fig. 2e we plot the dependence of B W on the carrier density, extracted from the high-field Hall slope. This field increases with decreasing density and becomes immeasurably high when we approach the transition point. If we plot its inverse, 1/ B W , as a function of the density ( Fig. 2f ), we see that it extrapolates to zero at n C , the critical density that marks the onset of the observed transition. What is the nature of the observed transition point? Below V C ρ XY is linear with B , its slope is inversely proportional to V G , and ρ XX hardly changes with B , which is the classical behaviour expected from single-carrier transport. Above V C , on the other hand the S-shaped Hall traces and the strong positive magnetoresistance in ρ XX are suggestive of multi-carrier transport. Most studies so far focused on this high-carrier density regime, and interpreted the S-shaped Hall traces [11] , [12] , [19] , [22] to result from transport by two or more kinds of carriers. The transition that we observe in our measurement is therefore from one- to multiple-carrier transport, the latter being so far the more prevalent regime in studies of this system. The observation of a density regime in which transport is given by only a single-carrier type is in fact very surprising in light of the multitudinous d-bands predicted by theory [13] , [14] , and intimates that any additional bands that may exist in the system must have localized carriers that are irrelevant to transport. The simple generic form observed for the transport above V C suggests that even above V C the transport might be simpler than originally imagined. In fact it can be shown that the S-shaped transport traces above the transition point, as well as the observed correlation between ρ XY and ρ XX , could be nicely explained by a simple two-carrier transport model. A careful analysis of our data shows however that the transition field B W between one- and two-carrier transport is not accounted for by the simple two-carrier model, often used in the literature [24] , which assumes that the mobilities and densities of the two carriers are independent of magnetic field (described in Supplementary Methods ). We further show there that this assumption makes the simple model inadequate for extracting the two carrier mobilities, but that it can still reliably determine their densities. Specifically, if the two carriers have significantly different mobilities, the asymptotic value of R H at zero field gives the density of the high mobility carriers, n hi =1/ eR 0 , whereas its value at large fields yields the total density of both carriers, n total =1/ eR ∞ , ( e is the electron charge). In Fig. 3a we extract these two quantities, n hi and n total , from the Hall coefficients measured at B =0 T and 14 T , and plot them against V G . For voltages below the transition point we see that all the carriers are of the high mobility type, implied by the fact that n total ≈ n hi , and that their density is continuously tuned by the gate up to a critical value, n C . After crossing the transition point, n hi saturates at n C , whereas n total continues to rise, implying that at high densities only lower mobility carriers are added by the gate, in contrast to the notion that its main effect is to add carriers populating higher mobility TiO 2 planes at increasing distances from the interface. 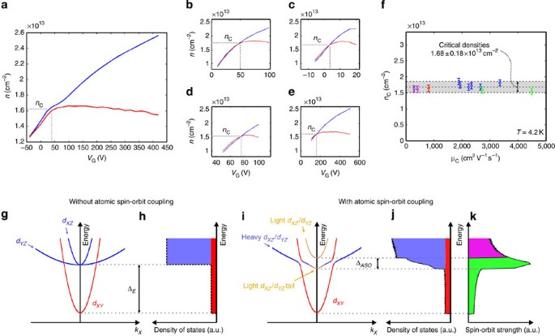Figure 3: Universality of the critical density and its energy bands origin. (a) Densities extracted from measured Hall coefficient (n=1/eRH,eis electronic charge) atB=0T(red) andB=14 T (blue) versusVG. The former reflects (see text) the density of high mobility carriers,nhi, and the latter the total density,ntotal. BelowVC(dashed vertical line),ntotal≈nhiand both increase withVGup to the critical value,nC, (dashed horizontal line) reached atVC. AboveVC,nhisaturates whereasntotalcontinues to increase. The data shown are from a 6 u.c. sample grown atTgrowth=800 °C. (b–e) Similar analysis on additional samples differing by LAO layer thickness and growth temperatures. (b,c) 10 u.c.,Tgrowth=650 °C. (d) 10 u.c.,Tgrowth=800 °C. (e) 6 u.c.,Tgrowth=800 °C. (f) Collection of critical densities measured with several independent Hall bars on four samples (different colours), versus electron mobility, μC, at the critical density. These critical densities show a universal value,nC=1.68±0.18×1013cm−2, independent of mobility and LAO thickness. The key to the different colours is, sample 1: 6 u.c.,Tgrowth=800 °C (purple), sample 2: 9 u.c.,Tgrowth=800 °C (red), sample 3: 10 u.c.,Tgrowth=800 °C (green) and sample 4: 10 u.c.,Tgrowth=650 °C (blue). (g)d-Orbital energy bands of STO near its interface with LAO. ThedXYband is lower in energy by ΔEcompared with thedXZanddYZbands. (h) Schematic DOS versus energy. ThedXYband has approximately ten times smaller DOS (red) than combined DOS ofdXZanddYZbands (blue; see text). (i) Calculated band structure including ASO interactions. At the Γ point the bands split by ΔASO(see alsoSupplementary Fig. S3andSupplementary Methods). (j) Calculated DOS with ASO. The sharp jump of (h) is smeared over a ΔASOscale. (k) Strength of ASO, ‹L·S›, integrated over the Fermi surface of the first two bands and plotted versus energy (green). ASO is strongly peaked near the critical point. Shown in purple is the absolute value, in the third band, of ‹L·S› which has the opposite sign compared with the first two bands. Although ASO is also sharply peaked near the bottom of the third band, the Fermi energy is always below the bottom of this band for typical carrier densities. Figure 3: Universality of the critical density and its energy bands origin. ( a ) Densities extracted from measured Hall coefficient ( n =1/ eR H , e is electronic charge) at B =0 T (red) and B =14 T (blue) versus V G . The former reflects (see text) the density of high mobility carriers, n hi , and the latter the total density, n total . Below V C (dashed vertical line), n total ≈ n hi and both increase with V G up to the critical value, n C , (dashed horizontal line) reached at V C . Above V C , n hi saturates whereas n total continues to increase. The data shown are from a 6 u.c. sample grown at T growth =800 °C. ( b – e ) Similar analysis on additional samples differing by LAO layer thickness and growth temperatures. ( b , c ) 10 u.c., T growth =650 °C. ( d ) 10 u.c., T growth =800 °C. ( e ) 6 u.c., T growth =800 °C. ( f ) Collection of critical densities measured with several independent Hall bars on four samples (different colours), versus electron mobility, μ C , at the critical density. These critical densities show a universal value, n C =1.68±0.18×10 13 cm −2 , independent of mobility and LAO thickness. The key to the different colours is, sample 1: 6 u.c., T growth =800 °C (purple), sample 2: 9 u.c., T growth =800 °C (red), sample 3: 10 u.c., T growth =800 °C (green) and sample 4: 10 u.c., T growth =650 °C (blue). ( g ) d -Orbital energy bands of STO near its interface with LAO. The d XY band is lower in energy by Δ E compared with the d XZ and d YZ bands. ( h ) Schematic DOS versus energy. The d XY band has approximately ten times smaller DOS (red) than combined DOS of d XZ and d YZ bands (blue; see text). ( i ) Calculated band structure including ASO interactions. At the Γ point the bands split by Δ ASO (see also Supplementary Fig. S3 and Supplementary Methods ). ( j ) Calculated DOS with ASO. The sharp jump of ( h ) is smeared over a Δ ASO scale. ( k ) Strength of ASO, ‹ L·S ›, integrated over the Fermi surface of the first two bands and plotted versus energy (green). ASO is strongly peaked near the critical point. Shown in purple is the absolute value, in the third band, of ‹ L·S › which has the opposite sign compared with the first two bands. Although ASO is also sharply peaked near the bottom of the third band, the Fermi energy is always below the bottom of this band for typical carrier densities. Full size image An underlying universal Lifshitz transition How universal is the observed critical density? One expects that this density depends on the disorder and inhomogeneities in the system [4] , [9] , [25] , as well as on the different confinement potential profiles that can form at the interface. Indeed, for samples with low mobilities we find that the critical density can change substantially from sample to sample. The surprising observation is, however, that in all high mobility samples that we have measured we observe a striking universality in the critical density. In Fig. 3b–e, we show measurements on additional samples whose LAO layer thicknesses varied from 6 to 10 unit cells and whose mobilities varied by an order of magnitude, analysed like in Fig. 3a . In all cases, we observed similar Hall and longitudinal resistance traces and comparable transition points, where the transport switched from one to two kinds of carriers (see also Supplementary Fig. S1 ). Whereas the critical gate voltage and the mobility at the transition, μ C , vary substantially between samples, the critical density in these high mobility samples is almost the same. Plotting the critical density versus the critical mobility measured in several independent Hall bars on four different samples ( Fig. 3f ), we see that these densities have a universal value n C =1.68±0.18×10 13 cm −2 independent of disorder, pointing to an intrinsic origin. The observed critical density is therefore fundamentally different from the recently determined metal–insulator transition density [26] , both in its experimental signature (below the metal–insulator transition the I–V characteristics are non-ohmic, whereas we see ohmic behaviour throughout except at the lowest densities, which are much smaller than n C ), as well as in its underlying source: the metal–insulator transition density is non-universal [26] , being set by the extrinsic disorder, whereas the critical density that we observe is universal, pointing to an intrinsic source. We argue that the observed transition is a Lifshitz transition that occurs when the density exceeds a critical value at which new bands of a different symmetry are populated. It is well established that interfacial electrons reside in the t 2g conduction bands of STO [27] , [28] , [29] , [30] . In the bulk, these three bands are degenerate, having ellipsoidal Fermi surfaces centered at the Γ point and oriented along the main lattice directions. At the interface this degeneracy is lifted due to tetragonal distortion and quantum confinement. Specifically, the d XY band, which has a larger effective mass in the z-direction than the d XZ and d YZ bands, splits toward lower energy [27] ( Fig. 3g ). Therefore, below a critical carrier density all electrons are expected to reside in the d XY band and only one type of carrier exists in the system. At higher densities the Fermi energy enters the d XZ and d YZ bands, and as they both get populated we expect to observe contributions from carriers of a new type. The Lifshitz transition into the new bands is accompanied by a large change in the density of states (DOS), determined by the geometric mean of the effective masses in the 2D plane, . As the d XZ and d YZ bands each has one light and one heavy mass in the plane whereas the d XY band has two light masses, the latter has the lowest DOS ( Fig. 3h ). Using effective masses determined from angle-resolved photoemission spectroscopy [28] , the combined DOS of the d XZ and the d YZ bands is approximately ten times higher than that of d XY band. Therefore, after raising the Fermi energy above the critical density, we expect the two newly occupied heavy bands to take up most of the added carriers while the density of the light d XY carriers remains almost constant. This scenario perfectly fits our observations plotted in Fig. 3a–e and excludes the possibility of an upper band being a more mobile, sub-band replica with the same symmetry as the lower band. The effect of SO coupling on the band structure ( Fig. 3i–k ) is discussed below. We can now address the observed universality of the critical density. Within the above band model, the critical density is determined by the number of carriers that the d XY band can accommodate before the higher bands become available, . Here, Δ E is the energy splitting between the d XY and the higher two bands, and m l is the light mass. Using the X-ray measured splitting [27] , Δ E =50 me V, and angle-resolved photoemission spectroscopy measured light mass [28] , m l =0.7 m e ( m e is the electronic mass), we estimate that n C =1.46×10 13 cm −2 , in good agreement with our experimentally determined value of n C =1.68±0.18×10 13 cm −2 . In general, Δ E can have non-universal contributions from gate-induced electric fields, the nonlinear dielectric constant of STO and charge traps, and a universal contribution from a charge or a dipole layer at the LAO/STO interface, as implied by recent measurements [31] . Our observation of a universal transition density suggests that an intrinsic mechanism, such as the proposed dipole layer, is the dominant component of the confinement potential at the interface ( Supplementary Discussion ). The body of evidence presented above lends strong support to the interpretation that the observed Lifshitz transition occurs when d-bands of a different symmetry begin to be populated. It is interesting to see how this physics comes to bear on superconductivity in the system. 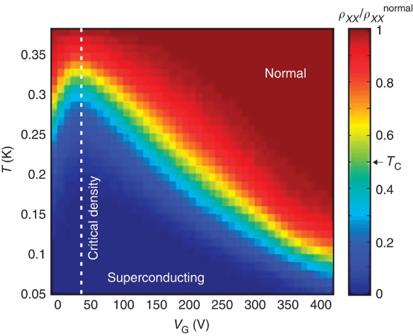Figure 4: Correlation between superconductivity and the critical density. ρXXmeasured versus temperature and gate voltage, divided by its normal-state value atT=0.38 K. Red and blue colours correspond to the normal and superconducting states. The superconducting transition temperature,TC, defined by, has a dome shape as function ofVG. The critical density (white dashed line) is found to be at the peak of the dome. Figure 4 shows the longitudinal resistivity ρ XX measured down to T =50 mK, divided by its normal-state value at T =0.38 K, as a function of temperature and gate voltage. As reported earlier [6] , [7] , [10] , [11] , we find that superconductivity is dome-shaped as a function of V G . The superconducting transition temperature, T C , first increases rapidly with V G up to a peak value, T C max =320 mK, after which it slowly decreases with increasing V G . Comparing these measurements to the critical density (dashed line in Fig. 4 ), we find that the latter corresponds to the peak of the dome. A similar correlation could also be deduced for published data [11] if we apply to it the analysis described above. Although the full details of 2D superconductivity in this system are still not fully understood the observed correlation hints that the Lifshitz transition is probably having an important role in this phenomenon. Figure 4: Correlation between superconductivity and the critical density. ρ XX measured versus temperature and gate voltage, divided by its normal-state value at T =0.38 K. Red and blue colours correspond to the normal and superconducting states. The superconducting transition temperature, T C , defined by , has a dome shape as function of V G . The critical density (white dashed line) is found to be at the peak of the dome. Full size image We now turn to discuss how the band picture that emerges from our experiments can readily explain the strong gate tunability of SO interactions observed in previous experiments. Earlier transport measurements [10] have used weak anti-localization analysis to show that the strength of SO interactions rises sharply at a certain gate voltage, concomitant with the rise of T C . Measurements of the superconducting critical field [12] have further indicated that at higher gate voltages, SO interaction strength reduced gradually. So far, the existence of SO in this system has been explained to result from Rashba interactions that are induced by the electric field of the confining potential [10] , [12] , [17] . However, in a simple Rashba picture it is unclear why SO will suddenly increase at a certain density, nor why similar SO effects are observed in δ-doped STO [32] , whose confining potential is symmetric. We argue that the observed dependence of SO on the carrier density can be naturally understood within the band picture discussed above. The key is to realize that the strongest SO effect in this system is the atomic SO (ASO) coupling [33] , [34] . ASO is especially prominent when the d-bands are degenerate, so that the coupling strongly mixes the orbitals and entangles the spin and orbital degrees of freedom [35] . When we add ASO to the band calculation ( Fig. 3i,j ), we indeed see that its most marked effect is near the bottom of the d XZ and d YZ bands. Interestingly, we find that the calculated ASO strength as a function of energy ( Fig. 3k , see caption for details) peaks around the transition point in a striking resemblance to the experimental observation [10] , suggesting that intrinsic ASO at the band transition is responsible for the strong SO observed in this system. We note that other band-structure effects could also mix the d XZ and d YZ bands, where the leading contribution, not excluded by symmetry, is due to second-nearest neighbour hopping between d XZ and d YZ orbitals along a diagonal. However, unlike ASO, which mixes the bands even at the Γ point, the diagonal hopping is proportional to the crystal momentum squared and thus is very small around the Lifshitz transition at the Γ point. In the Supplementary Methods (see also Supplementary Fig. S2 ), we estimate the strength of the diagonal hopping by fitting a tight binding model to density functional theory calculations without ASO [13] , and show that its inclusion in our Hamiltonian has negligible effects on the band-structure in the relevant energy window around the Lifshitz point ( Fig. 3i–k ). We further show how the intimate connection between the Lifshitz transition and ASO may also explain other observations in this system, most notably the low-carrier densities measured by Shubnikov–de Haas [18] , [19] , [36] , [37] , [38] . The Rashba SO coupling existing in this system is intimately tied to its strong ASO coupling. Microscopically, Rashba coupling emerges as a second-order perturbation in ASO when the inversion symmetry of the interface is broken (more details in Supplementary Methods ). This coupling is therefore directly proportional to the strength of ASO and thus its strength will also peak at the Lifshitz point. In the presence of such coupling, the anisotropy of transport with in-plane magnetic field [39] can serve as a probe of the orbital symmetry of the conduction bands [40] . Our recent measurements of this anisotropy not only indicate the buildup of SO coupling when the Lifshitz transition is approached from above but also show that below the critical density the system has an isotropic ground state, consistent with a circular d XY band, whereas above it the ground state acquires a strong crystalline anisotropy, consistent with the elliptical d XZ and d YZ bands that are oriented along the crystalline directions [41] . In summary, we observe that the 2D system formed at the LAO/STO interface undergoes a Lifshitz transition, which reshapes its core transport properties above a critical carrier density. The value of the critical density is observed to be universal, independent of sample mobility and LAO layer thickness. This transition is understood to be between d XY and d XZ / d YZ orbital population, showing that out of the multitude of d-bands predicted theoretically, only a small subset is relevant to fully capture the physics of the conducting 2D system. We show that near the transition ASO interactions should become prominent, accounting for the peak of SO strength observed experimentally. We further observe a similar correlation between this transition and the peak of superconducting T C , which may suggest that the population of the d XZ and d YZ bands at this critical density has an important role in the emergence of superconductivity as well as possibly other correlated states in this system. These results therefore open the way to a fundamental description of the fascinating behaviours of this system in terms of an underlying, universal transition between states of different orbital symmetries. Sample fabrication As detailed in an earlier work [6] , LaAlO 3 films were grown on TiO 2 -terminated (001) SrTiO 3 single crystals by pulsed laser deposition in ~10 −4 mbar of O 2 . The repetition rate of the laser was 1 Hz, with the fluence of each pulse being 0.6 J cm −2 . The film growth was monitored in situ using reflection high-energy electron diffraction. Three samples were grown at T =800 °C and the last at T =650 °C to yield higher mobility [18] . After growth, the samples were annealed in 200 mbar of O 2 at about 600 °C for 1 h and cooled to room temperature in the same oxygen pressure. For the high mobility sample, annealing took place at 530 °C. More information including the influence of oxygen pressure during growth can be found in Cancellieri et al . [42] Hall bars were photolithographically patterned and the sample was ultrasonically bonded using Al wire. Measurement Transport was measured using standard back-gated Hall bars with widths varying from 100 to 500 μm and AC currents of 5–50 nA. In the entire range of gate voltages studied the measured resistance was ohmic. Most measurements were done at T =4.2 K, apart from those of superconductivity that were done down to 50 mK. The longitudinal (Hall) resistivity was symmetrized (anti-symmetrized) with respect to magnetic field to eliminate small spurious effects from lithographic imperfections. How to cite this article: Joshua A. et al . A universal critical density underlying the physics of electrons at the LaAlO 3 /SrTiO 3 interface. Nat. Commun. 3:1129 doi: 10.1038/ncomms2116 (2012).